Experimental loss-tolerant quantum coin flipping Coin flipping is a cryptographic primitive in which two distrustful parties wish to generate a random bit to choose between two alternatives. This task is impossible to realize when it relies solely on the asynchronous exchange of classical bits: one dishonest player has complete control over the final outcome. It is only when coin flipping is supplemented with quantum communication that this problem can be alleviated, although partial bias remains. Unfortunately, practical systems are subject to loss of quantum data, which allows a cheater to force a bias that is complete or arbitrarily close to complete in all previous protocols and implementations. Here we report on the first experimental demonstration of a quantum coin-flipping protocol for which loss cannot be exploited to cheat better. By eliminating the problem of loss, which is unavoidable in any realistic setting, quantum coin flipping takes a significant step towards real-world applications of quantum communication. Coin flipping is the art of tossing a coin to allow two parties to choose between two alternatives in the least biased way. The importance of this primitive led Manuel Blum to introduce 'coin flipping by telephone', in which the two spatially separated parties do not necessarily trust each other but still wish to ensure that the outcome of the coin flip is unbiased [1] . Throughout this article, we only consider asynchronous protocols, which consist of a sequence of rounds in which Alice and Bob alternate in sending classical or quantum messages to each other. For any such classical coin-flipping protocol, one of the parties can, given sufficient computational power, deterministically choose the outcome, in which case we say the protocol is broken. In the quantum world, this is no longer true [2] , [3] , [4] , [5] , [6] . Although no unbiased protocol can exist [7] , [8] , the probability for a cheater to fix an arbitrary desired outcome can be asymptotically reduced [9] to (the possibility that a cheater may be interested in obtaining either outcome defines strong coin flipping; the only type of protocols considered here). This bound is due to Kitaev [9] , whose proof is reproduced in ref. 10 . Note that quantum coin flipping differs from quantum key distribution [11] , [12] in the fact that Alice and Bob are potential adversaries, not collaborators. The importance of quantum coin flipping lies not only in its potential for applications, but also, more fundamentally, in the fact that quantum communication allows one to implement a cryptographic primitive that is impossible using solely classical communication. The typical structure of most previous protocols is as follows. Alice sends a quantum state | ψ > to Bob, chosen from an agreed-upon set, that conceals a bit a . Bob returns a classical bit b . Alice then discloses which | ψ > was sent, thereby revealing a . Bob can now perform a measurement on the received state, the result of which should confirm that Alice did indeed send state | ψ >. If Bob's result is inconsistent with the description | ψ >, he declares a mismatch. Otherwise, the outcome c of the coin flip is the exclusive OR of a and b , denoted c = a ⊕ b . Importantly, Alice must not be able to declare a value of a that depends on the value of b without risking being caught cheating through Bob's measurement of | ψ >. Furthermore, Bob must not be able to determine the value of a from a measurement of | ψ > before returning his bit. As usual in quantum communication, quantum states are encoded into photons, which are susceptible to loss in the transmission channel and measurement apparatus. For quantum coin flipping, the mere possibility that Bob may not detect Alice's quantum state can be highly problematic [13] , [14] . For example, if the protocol specifies that Bob's measurement happens after Alice revealed her bit, this allows him to cheat by pretending that the quantum state was lost whenever he is not happy with a ⊕ b . Consequently, if Alice allows the protocol to be restarted until Bob declares a detection, the latter can completely control the outcome. Unfortunately, this practical problem has been overlooked in almost all previous protocols [2] , [3] , [4] , [5] , [6] . Therefore, any implementation based on such protocols is completely broken under realistic experimental conditions. Before this work, two quantum coin-flipping protocols have been implemented. The first implementation [15] is based on a protocol that is completely broken in the presence of loss [14] . The second avoids this pitfall by using a protocol that does not require Bob to detect a photon to produce an outcome [16] . This, however, gives rise to a new attack in which a malicious Alice tampers with the loss of the transmission line, such that her probability to choose the outcome is arbitrarily close to 100%, which makes this protocol effectively broken. In the reported implementation of this protocol, Alice could choose the outcome with a probability of 99.71% for 16 dB loss. This probability would further increase for higher loss. Therefore, both aforementioned protocols, and their implementations, could hardly (if at all) be used in any practical application based on coin flipping. To be of practical use, a protocol should be designed to tolerate loss in the transmission channel. Here we present the first experimental demonstration of a quantum coin-flipping protocol for which loss cannot be exploited to cheat better. More precisely, our implementation allows us to bound the successful cheating probability to a value that is independent of loss. A loss-tolerant quantum coin-flipping protocol We begin with describing our protocol. We refer to our original proposal for a thorough description [14] . Let us first assume that both parties are honest. Alice sends a qubit whose state | ψ x , a > is chosen randomly among the following, previously agreed-upon set ( Fig. 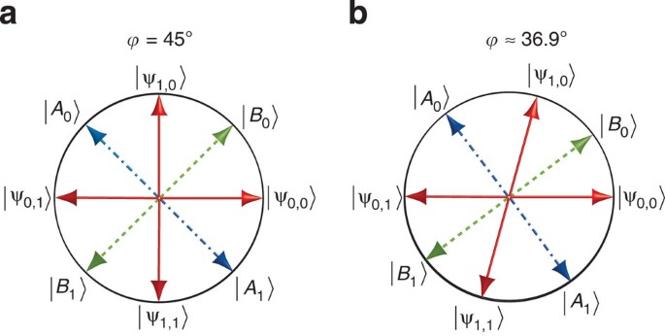Figure 1: Honest and cheating states of the loss-tolerant protocol. The states used are represented on a great circle on the Bloch sphere. (a) BB84 states, corresponding cheating states |A0> and |A1> for Alice, equal towithϕA=67.5°, and corresponding cheating states |B0> and |B1> for Bob, equal towithϕB=22.5°. (b) Fair states and the corresponding cheating states defined as for the BB84 states but withϕA≈63.4° andϕB≈18.4°. 1 ): Figure 1: Honest and cheating states of the loss-tolerant protocol. The states used are represented on a great circle on the Bloch sphere. ( a ) BB84 states, corresponding cheating states | A 0 > and | A 1 > for Alice, equal to with ϕ A =67.5°, and corresponding cheating states | B 0 > and | B 1 > for Bob, equal to with ϕ B =22.5°. ( b ) Fair states and the corresponding cheating states defined as for the BB84 states but with ϕ A ≈63.4° and ϕ B ≈18.4°. Full size image where | ϕ + >=cos ϕ |0>+sin ϕ |1>, | ϕ − >=sin ϕ |0>−cos ϕ |1> and 0°< ϕ ≤45°. Here we call x and a Alice's basis and bit , respectively. Bob then attempts to measure Alice's qubit in a basis y ∈ {0,1} from the set described above, chosen at random. If Bob does not detect the qubit, he asks Alice to send another randomly selected state. This is repeated until Bob detects the qubit, in which case he sends a random bit b to Alice. When Alice receives b , she reveals x and a to Bob. If y = x , Bob's measurement outcome should agree with Alice's declared state | ψ x , a >, in which case a is accepted. In case of a disagreement, Bob declares a mismatch. If y ≠ x , Bob has no way to verify Alice's claim and he must accept her bit on faith. The outcome of the protocol is c = a ⊕ b . Note that we do not consider denial-of-service attacks, as in the case where Bob postpones the outcome of a coin flip indefinitely. The loss tolerance of our protocol stems from two features. The first is that Bob's declaration of a successful measurement happens before Alice reveals her bit a . The second is that Bob gains no advantage in falsely declaring that Alice's qubit was lost. In particular, it is physically impossible for Bob to conclusively determine Alice's bit a with certainty, given a single copy of | ψ x , a >. The performance of optimal cheating strategies depends on the value of ϕ . For the states given in equation (1) with ϕ =45°, which we refer to as the BB84 states ( Fig. 1a ), Alice's maximum probability to fix the outcome, P A , is she is caught cheating with the complementary probability, that is, when a mismatch occurs. Bob's equivalent probability, , which makes the use of these symmetrically distributed states unfair as Alice can cheat better. By setting ϕ =arccos(4/5) ∼ 36.9°, which results in what we call the fair states ( Fig. 1b ), this asymmetry is removed, leading to P A = P B =90%. For both sets of states, Alice's optimal cheating strategy consists of randomly sending one of the two orthogonal states | A 0 > and | A 1 > that are positioned symmetrically between states representing different bit values a , as shown in Figure 1 . This choice allows her to always declare an x and a that will produce the outcome of her choice while minimizing her probability of being caught cheating. Bob's optimal cheating strategy consists of measuring the received qubit in basis {| B 0 >,| B 1 >}, where | B i > is positioned symmetrically between the states that correspond to the bit value a = i , as shown in Figure 1 . This maximizes his probability to guess the value of Alice's bit. We do not consider the case in which both Alice and Bob are cheating, as the goal of the protocol is to protect honest players only. So far, we considered the noiseless scenario in which declaration of a mismatch occurs only if a player is trying to cheat. In general, however, the presence of intrinsic noise entails a probability of getting a mismatch as the outcome, even if both players are honest. Nevertheless, the cautious honest player should assume the declaration of a mismatch to be due to cheating, and not allow restarting the protocol in this case. Hence, the ideal scenario can be approximated only if the intrinsic noise level is small. We stress, however, that the presence of noise has no effect on the key property of our protocol and implementation, namely that P A and P B are upper bounded independently of loss. This makes quantum coin flipping possible in the presence of loss. Experimental set-up For the experimental implementation of the protocol, the restrictions on Alice's qubit source are very stringent, even more than in quantum key distribution, as Bob is an adversary who is potentially cheating. With current technology, one practical choice is to use a suitably designed source of pairs of entangled qubits such that projecting one qubit at Alice's remotely prepares the qubit sent to Bob in a state chosen at random among the states of equation (1). We already presented a security proof in the case where Alice sends qubits encoded into true single photons and where the experiment is noiseless [14] . A complete security proof for an implementation based on a source of entangled photons should, however, take into account all possible sources of imperfections and possibly requires adapting squashing models developed for some quantum key distribution protocols [17] , [18] (see Methods). We note that because of the adversarial nature of Alice and Bob, and the particular choice of projection measurements, these studies do not straightforwardly apply to our coin-flipping protocol. 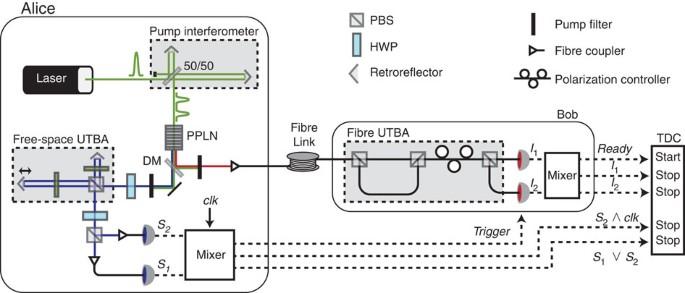Figure 2: Experimental set-up. A laser diode sends 50 ps pulses at 530.6 nm wavelength through an interferometer with path-length difference equivalent to 1.4-ns travel-time difference. The pulses emerge in an even superposition of two well-defined time bins that we label the early and late bins and then propagate into a nonlinear, periodically poled lithium niobate crystal (PPLN), thereby creating time-bin entangled qubits at 807 and 1,546 nm wavelengths through spontaneous parametric downconversion. The two qubits are separated at the dichroic mirror (DM). The free-space and fibre UTBAs allow Alice and Bob to measure their qubits in randomly selected basesxandy, respectively, as defined by equation (1); see Methods. The angleϕis selected by the orientation of the output half-wave plate (HWP) at Alice's and the polarization controller at Bob's. The coincidence detections are monitored using a TDC and analysed in real-time to realize all steps of the protocol. Clk; laser clock; PBS, polarization beam splitter. Our experimental set-up is detailed in Figure 2 . Time-bin entangled photonic qubits [19] in the state Figure 2: Experimental set-up. A laser diode sends 50 ps pulses at 530.6 nm wavelength through an interferometer with path-length difference equivalent to 1.4-ns travel-time difference. The pulses emerge in an even superposition of two well-defined time bins that we label the early and late bins and then propagate into a nonlinear, periodically poled lithium niobate crystal (PPLN), thereby creating time-bin entangled qubits at 807 and 1,546 nm wavelengths through spontaneous parametric downconversion. The two qubits are separated at the dichroic mirror (DM). The free-space and fibre UTBAs allow Alice and Bob to measure their qubits in randomly selected bases x and y , respectively, as defined by equation (1); see Methods. The angle ϕ is selected by the orientation of the output half-wave plate (HWP) at Alice's and the polarization controller at Bob's. The coincidence detections are monitored using a TDC and analysed in real-time to realize all steps of the protocol. Clk; laser clock; PBS, polarization beam splitter. Full size image are created, where | e > A ( B ) and | ℓ > A ( B ) represent the early and late time-bin states of Alice (Bob) and are associated with the generic states |0> and |1> used above to describe the protocol. One qubit remains in Alice's laboratory where it is randomly projected on one of the four states defined in equation (1) using a universal time-bin qubit analyser [20] (UTBA); see Methods for details. This has the effect of remotely preparing the other qubit in the same state. The latter is sent to Bob over the quantum channel consisting of 10 m polarization-maintaining fibre (this short link was later replaced by a 12.4 km underground fibre link; see below). The total photon loss of the 10 m link, which includes the coupling of Bob's photon into the optical fibre, all optical losses and the inefficiency of Bob's detectors, was equal to 23.2±2.0 dB. Bob, by virtue of his UTBA, then measures his time-bin qubit in a randomly chosen basis y . The UTBAs enable projective measurements of time-bin qubits in arbitrary bases, which facilitates the implementation of the fair protocol and of all the cheating strategies. Each coincidence detection between Alice and Bob defines a coin-flip instance for which all steps of the protocol are performed as described above. Therefore, each instance is a complete demonstration of our protocol. Performance of loss-tolerant quantum coin flipping We performed coin flipping both with the BB84 and the fair states, in each case with honest players or one cheater, as determined by the settings of the UTBAs. For each configuration, we performed at least 80,000 instances over the 10 m link. Let us consider the honest cases first. We estimated the intrinsic error probability P * , that is the probability for Bob to declare a mismatch when nobody is cheating, and the probabilities P 0 and P 1 of outcomes c =0 and 1 per coin-flip instance. 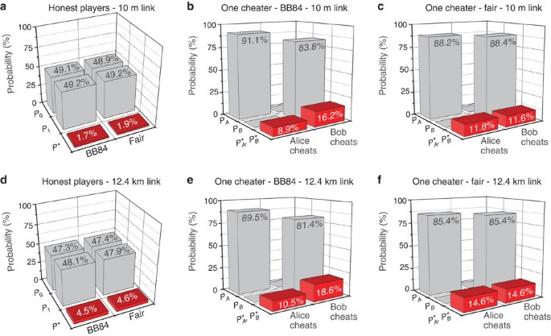Figure 3: Results. The column plots show the honest-player cases (a,d), one-cheater cases with BB84 states (b,e) and the one-cheater cases with fair states (c,f). All data collection runs consisted of at least 80,000 (or 7,000) coin-flip instances with the 10 m link (or the 12.4 km link); the one-standard-deviation uncertainties onP0,P1,PAandPBare at most 0.15% (or 0.5%); the uncertainty onP*is at most 0.04% (or 0.1%); the uncertainties onPA* andPB* are at most 0.13% (or 0.5%). All uncertainties are statistical assuming a Poisson distribution. As shown on Figure 3a , the P * obtained when using either the BB84 or the fair states is less than 2%, and the outcome probabilities P 0 and P 1 are equal within one standard deviation. The non-zero P * is caused by intrinsic noise stemming from experimental imperfections. Figure 3: Results. The column plots show the honest-player cases ( a , d ), one-cheater cases with BB84 states ( b , e ) and the one-cheater cases with fair states ( c , f ). All data collection runs consisted of at least 80,000 (or 7,000) coin-flip instances with the 10 m link (or the 12.4 km link); the one-standard-deviation uncertainties on P 0 , P 1 , P A and P B are at most 0.15% (or 0.5%); the uncertainty on P * is at most 0.04% (or 0.1%); the uncertainties on P A * and P B * are at most 0.13% (or 0.5%). All uncertainties are statistical assuming a Poisson distribution. Full size image Next, we consider the cases in which either Alice or Bob tries to fix the outcome c of every coin flip. The cheater's UTBA was aligned for optimal cheating. For each instance, the cheater chooses a desired value for c , uniformly distributed. We experimentally estimated the probability P A ( P B ) for Alice (Bob) to fix the outcome to the desired bit value, as well as P A * ( P B *), the probability of a mismatch in the presence of cheating. We assumed that a cheating Bob would always declare a mismatch when he was unhappy with the outcome. Therefore, P A + P A * = P B + P B * = 1. As a first observation of the results presented in Figure 3b , we note that the values obtained for P A and P B with the BB84 states are clearly unfair as P A > P B , in full accordance with the theory. In Figure 3c , we see that this asymmetry is removed when using the fair states. Furthermore, when using the BB84 states, P A =91.1±0.1%, which is higher than 90% by 11 standard deviations, that is, we are able to show that Alice can significantly cheat better than what is theoretically possible with the fair states. Similarly, when using the fair states, P B =88.4±0.1%>85.4% by 30 standard deviations, which demonstrates that Bob can significantly cheat better than what is theoretically possible with the BB84 states. Finally, we note that the probability for a mismatch to occur increases from P * <2% to P A *, P B * ≥ 8.9% in the presence of optimal cheating. To test our set-up in a real-world setting, we replaced the 10-m link with a 12.4 km long underground standard telecommunication fibre link connecting two laboratories positioned at the University of Calgary (UofC) and at the Southern Alberta Institute of Technology (SAIT), respectively. In particular, this allowed us to study the effect of loss on the performance of our implementation. The two locations are physically separated by 3.3 km and the total photon loss was equal to 32.8±2.0 dB. The modifications to the set-up required to realize the experiment over the underground fibre link are detailed elsewhere [20] . Globally, the effect of the added loss is to decrease the signal-to-noise ratio and, consequently, to increase the error probabilities P * , P A * and P B * and lower all other probabilities ( Fig. 3d–f ). We stress that this is due to the presence of experimental imperfections, such as detector dark counts, and not because of the protocol itself. Moreover, as discussed below, this could be mitigated with state-of-the-art single-photon detector technology. Quantum coin flipping in the presence of noise To gain further insight into how noise affects an implementation of our protocol when based on a source of entangled photons, we modelled the detection statistics of such an implementation taking into account loss, detector dark counts, multi-pair emission and imperfect optical alignment ( Supplementary Notes 1–3 ). 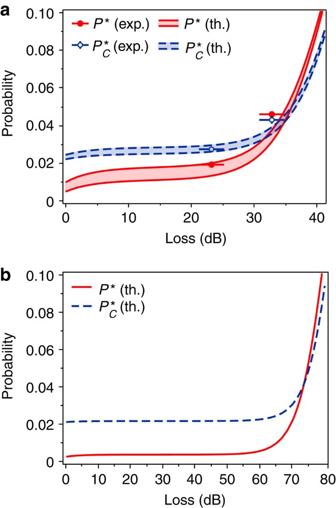Figure 4: Performance with varying loss with the fair states. (a) The experimentally measured values of the intrinsic error probabilityP*(solid circles) and the theoretically calculated values, using the estimated experimental parameters (shaded area, delimited by solid lines) as a function of the total loss of Bob's photon. The parameters are the mean number of photon pairs generatedμ, the transmission of Alice's channelηA, the probability of a dark count per 400-ps detection window for Alice's (Bob's) detectorsdA(dB), and the fidelityFof the generated entangled state with respect to state |Φ+>. We usedμ=0.032±0.004,ηA=7.56±2.23%,dA=4×10−8,dB=2.5×10−5,F=97.8±0.3% (Supplementary Table S1). Also shown are the values ofPC* (hollow circles) corresponding to our measured values ofPAandPB, as well as the theoretically calculated values (shaded area delimited by dashed lines). (b) Theoretically calculated values ofP*(solid line) andPC* (dashed line) as a function of the total loss of Bob's photon assuming ultra-low-noise detectors for Bob, that is,dB=10 Hz×400 ps=4×10−9, and slightly improved experimental conditions, that is,μ=0.005,ηA=9.8%,dA=4×10−8,F=99.25%. Using our estimated experimental parameters, we produced a theoretical curve of the intrinsic error probability P * as a function of the total loss applied to Bob's photon, and compared it against the measured values with the fair states; Figure 4a . The model compares well with the measurements. The model predicts that P * should equal 10% in the vicinity of 40 dB loss. With this model, we can also directly show that the increase of P * originates mostly from dark counts at Bob's detectors. This becomes clear when considering Figure 4b showing the theoretical curve of P * (solid line) generated assuming a dark count rate of 10 Hz for Bob's detectors, as well as slightly improved experimental conditions. Note that noise-free single-photon detectors at 1,550 nm have been reported [21] , making our assumption realistic. Under these conditions, and for loss up to 50 dB, P * is essentially constant. Moreover, the low value of P * one would obtain ( ∼ 0.37%) highlights that the transmission and measurement of photonic qubits is much more likely to be affected by loss than by noise. This shows the need for a protocol to tolerate loss. Figure 4: Performance with varying loss with the fair states. ( a ) The experimentally measured values of the intrinsic error probability P * (solid circles) and the theoretically calculated values, using the estimated experimental parameters (shaded area, delimited by solid lines) as a function of the total loss of Bob's photon. The parameters are the mean number of photon pairs generated μ , the transmission of Alice's channel η A , the probability of a dark count per 400-ps detection window for Alice's (Bob's) detectors d A ( d B ), and the fidelity F of the generated entangled state with respect to state |Φ + >. We used μ =0.032±0.004, η A =7.56±2.23%, d A =4×10 −8 , d B =2.5×10 −5 , F =97.8±0.3% ( Supplementary Table S1 ). Also shown are the values of P C * (hollow circles) corresponding to our measured values of P A and P B , as well as the theoretically calculated values (shaded area delimited by dashed lines). ( b ) Theoretically calculated values of P * (solid line) and P C * (dashed line) as a function of the total loss of Bob's photon assuming ultra-low-noise detectors for Bob, that is, d B =10 Hz×400 ps=4×10 −9 , and slightly improved experimental conditions, that is, μ =0.005, η A =9.8%, d A =4×10 −8 , F =99.25%. Full size image The presence of noise has another consequence on implementations of coin-flipping protocols. For given values of P 0 , P 1 , P * , P A ≥1/2 and P B ≥1/2, it was recently reported [22] (see also ref. 16 ) that there exist classical protocols yielding this set of probabilities if and only if P 0 , P 1 ≤ P A P B and This defines a benchmark for comparison between a noisy implementation of a quantum protocol and what is classically possible, as proposed in ref. 16 . Specifically, assuming P 0 , P 1 ≤ P A P B holds, one can define a figure of merit M = P C * − P * that is zero or negative if, and only if, there exists a classical protocol capable of reproducing the results. The first implementation yielding a positive M was reported in ref. 16 , but it remains of limited interest because it is effectively broken in the presence of loss. As shown in Table 1 , our results over the 10 m link yield a positive M and, therefore, cannot be reproduced classically. For the 12.4 km link, M lies around zero with the fair states (considering uncertainty), meaning that our implementation performs neither better nor worse than what is classically possible. This is consistent with the predictions of our model of the detection statistics ( Fig. 4a ). With the BB84 states, however, we obtain M <0, which means that our results could be reproduced classically. For completeness, we point out that the P C * one could expect using ultra-low-noise detectors at Bob's is well above P * (dashed line on Fig. 4b ). Table 1 Figure of merit. Full size table The work presented here shows how the problem of loss, the prominent issue plaguing previous protocols and implementations, can be alleviated using a suitably designed protocol. During the preparation of this work, other groups have shown that our protocol can be modified to reduce the bias slightly [23] , [24] . Alternatively, a device-independent and loss-tolerant protocol, having a bias lower than our protocol, was recently proposed [25] . Whether a loss-tolerant protocol can asymptotically reach the optimal bound for strong coin flipping [9] is still an open question. Experimental noise can never be completely eliminated, and one must always compare the performance of a noisy implementation of a loss-tolerant protocol to classical protocols, as we have done here. It is not known if a noise-tolerant protocol, that is a protocol such that P * =0 despite experimental imperfections [14] , can exist. In the negative, one could envision other (classically impossible) tasks that are based on repeated executions of our protocol. As suggested previously [13] , [26] , those tasks might benefit from the cheat sensitivity of our protocol. Our work also raises the question of whether sophisticated approaches developed to prove the security of practical implementations of quantum key distribution, such as a squashing model, can be adapted to scenarios where both parties are distrustful of each other. This largely unexplored theme is of central importance for the security of two-party cryptographic protocols based on imperfect devices. Source of entanglement The pump laser was operated at a repetition rate of 10 MHz ( Fig. 2 ). The 10-mm long periodically poled lithium niobate crystal, with a 7.05-μm grating period, was heated to 176 °C. The mean number of photon pairs created per pump pulse was about 0.05, which sets the probabilities to create one and two pairs to 4.8% and 0.12%, respectively [27] . The created state is very close to being maximally entangled [20] . The observed noise comes mostly from dark counts in Bob's InGaAs detectors and from imperfect optical alignment of the bulk interferometers. Detection events were acquired by a time-to-digital converter (TDC), which measures delays between a start signal and several stop signals. The detection signals from Alice's free-running Si-based single-photon detectors were preprocessed with an electronic mixer ( Fig. 2 ). The trigger signal was generated when a detection at either S 1 or S 2 occurred. It emerged synchronously with the laser clock ( clk ). The signal was used to gate Bob's InGaAs-based single-photon detectors during a 7-ns activation window. The signal ready , which was emitted only when both detectors were ready to detect, was used to start the TDC. This ensures that the statistics were not biased by the dead-time of Bob's detectors. The detections at I 1 and I 2 , as well as the signal S 2 clk and S 1 S 2 served as stop signals, where denotes the logical AND and the logical OR. This allowed us to register all possible coincidence detection events, where the detection slots, early, middle and late, were narrowed down to widths varying from 400 to 800 ps. This particular event selection to retrieve information about detections at S 1 and S 2 was chosen because of hardware considerations in Alice's mixer. Requirements on Alice's source of qubits The adversarial nature of the players forces Alice to consider side channels that a cheating Bob could exploit. For instance, when using attenuated laser pulses or a heralded single-photon source [28] , Alice will sometimes send multiple photons. In this case, all photons would be prepared in the same qubit state | ψ x , a >. In the presence of loss, this allows a cheating Bob to declare that the photon was lost unless he detects two photons in different bases using his honest measuring apparatus. When this happens, Bob can conclusively determine Alice's bit 64% of the time (with the fair states), in which case only will he declare the photon detected, thereby completely breaking the protocol [14] (however, see ref. 29 for an alternative approach based on our protocol that avoids this problem, but at the expense of losing loss tolerance). The ideal solution would be for Alice to use a perfect source of single photons, but this is not practical with current technology. A more realistic choice is to use a source of maximally entangled pairs of photonic qubits that are separated and directed to Alice and Bob, respectively. A projection measurement at Alice's then remotely prepares a state on Bob's photon [30] . To thwart potential attacks in which a malicious player exploits the fact that the (necessarily imperfect) source sometimes emits more than one photon pair, the honest players proceed as follows: first, Alice's source of entangled photons must be operated in the regime where the pump pulse duration ( T p ) is much longer than the coherence time ( τ c ) of the emitted photons. This condition, satisfied in our experiment (here, T p / τ c ≈185), ensures that all photon pairs generated by the same pump pulse are, with almost certainty, completely independent of each other. Second, Alice's basis choice must be passive so that each of Alice's photons is measured in an independently and randomly chosen basis. Third, both Alice and Bob (when honest) follow a procedure that is inspired by the squashing operation developed for projective measurements onto the BB84 states [17] , [18] . More precisely, in the eventuality of multiple simultaneous clicks, honest players privately choose, randomly and uniformly, one of the outcomes for completion of the protocol. The goal of this procedure is to render our overall set-up equivalent to the one in which only single pairs are created, and where the previously mentioned cheating attack does not exist [31] . While plausible, the possibility of generalizing the squashing model to our specific scenario, and, more generally, to scenarios involving two distrustful parties, is still an open question and its resolution is beyond the scope of this work. Universal time-bin qubit analysers The free-space UTBA shown in Figure 2 can be understood as follows [20] : the polarization of the incident time-bin qubit is first rotated to 45° with respect to the linear polarization transmitted by the input polarizing beamsplitter. After passing through an interferometer with large path-length difference, the qubit emerges in three chronologically ordered time slots separated by 1.4 ns that we label early, middle and late. In the middle slot, the initial time-bin qubit is mapped on a polarization qubit, which can be analysed in any basis using standard waveplates, a polarizing beamsplitter (PBS) and detectors. This implements the detection in the x =1 basis at Alice's, where the angle ϕ is determined by the orientation of the half-wave plate located at the output of the interferometer. This angle was calibrated independently and had an uncertainty of at most, 1°. A detection in the early (late) slots corresponds to a projection on | e > A (|ℓ> A ), and this implements a measurement in the x =0 basis. Therefore, the detection time at the single photon detectors S 1 and S 2 passively determines Alice's basis. This is similar to previous projection measurement schemes for time-bin qubits [32] , yet, without the restriction to mutually unbiased bases. Bob's fibre UTBA is the fibre-optics equivalent of Alice's free-space version. The input fibre, as well as the two arms of the interferometer, are made of polarization-maintaining fibre. The output of the interferometer is a standard fibre and the angle ϕ is selected by a polarization controller that was calibrated independently and had an uncertainty less than 2 degrees. Here again, the detection time at the single-photon detectors I 1 and I 2 determines Bob's basis. As both UTBAs are based on interferometers, they perform measurements in a given basis up to an azimuthal angle on the Bloch sphere. To implement the measurements needed to in the protocol, only the relative azimuthal angle between the bases of Alice and Bob's UTBAs matter. Hence, each data collection run started by an adjustment of the azimuthal angle of Bob's UTBA relative to Alice's, the latter being passively stabilized during data collection. Bob's angle was controlled using a circular piezo around which the fibre of the long arm was wound and glued. In this way, the angle could be selected with voltage. The relative angle was set to zero by maximizing the number of coincidences between I 1 and S 1 . This procedure also minimizes P * and maximizes P A and P B . The uncertainty on the values of ϕ of Alice's and Bob's UTBAs, as well as the relative azimuthal angle of their measurement bases, could have affected the performance of our implementation. However, because of the meticulous calibration of our UTBAs, the effect of systematic errors on the performance of our implementation is assumed to be negligible and was not included in the analysis. We note that, in principle, this assumption could be relaxed by using a device-independent quantum coin flipping protocol such as the one proposed recently in ref. 25 . How to cite this article: Berlín, G. , Brassard, G., Bussières, F., Godbout, N., Slater, J.A. & Tittel, W. Experimental loss tolerant quantum coin flipping. Nat. Commun. 2:561 doi: 10.1038/ncomms1572 (2011).